Magnetic flux lines in type-II superconductors and the 'hairy ball' theorem Many prominent phenomena originate from geometrical effects rather than from local physics. For example, the 'hairy ball' (HB) theorem asserts that a hairy sphere cannot be combed without introducing at least one singularity, and is fulfilled by the atmospheric circulation with the existence of stratospheric polar vortices and the fact that there is always at least one place on Earth where the horizontal wind is still. In this study, we examine the consequences of the HB theorem for the lattice of flux lines that form when a magnetic field is applied to a type-II superconducting crystal. We find that discontinuities must exist in lattice shape as a function of field direction relative to the crystal. Extraordinary, 'unconventional' flux line lattice shapes that spontaneously break the underlying crystal symmetry are thus remarkably likely across all type-II superconductors, both conventional and unconventional. A type-II superconductor responds to a moderate magnetic field by admitting the field as quantised lines [1] , each carrying flux Φ 0 = h /2 e . These lines nominally arrange in a two-dimensional lattice, with one Φ 0 per unit cell [2] . An equilateral triangular half-unit cell is expected in the isotropic case, but other shapes are frequently observed [3] , [4] , [5] , [6] , [7] , [8] , [9] , [10] , [11] and are usually interpreted in terms of anisotropies of the crystal or of the superconducting wave function. Hence, it is not surprising that, as one of the few probes of the superconducting state, the study of flux line lattice (FLL) shapes and orientations forms a cornerstone in our understanding of both conventional and unconventional superconductivity. In this study, we reveal that the occurrence of unusual FLL structures is rather likely for purely geometrical reasons, because the FLL must comply with the 'hairy ball' (HB) theorem [12] , [13] . We illustrate the remarkable, different ways in which this geometrical constraint may be fulfilled by considering the particular case of a superconducting niobium (Nb) crystal, though our arguments are general. For any superconductor, tuning the field value and temperature and varying the field direction may 'comb the HB' in a variety of different 'hairstyles'. The FLL may be imaged directly by neutron diffraction ( Fig. 1 ): the positions of the diffraction spots relative to the incoming beam give the lattice vectors (see Methods ). Within the superconductor, flux lines run parallel to the magnetic induction B . For a given B =| B |, the directions establish a sphere, and the lattice vectors of the FLL, tangent to the sphere, can be envisaged as 'hairs'. The HB theorem states that a continuous non-vanishing tangent vector cannot exist everywhere on a sphere. The original proof arises from the Poincaré–Hopf theorem [12] , [13] . 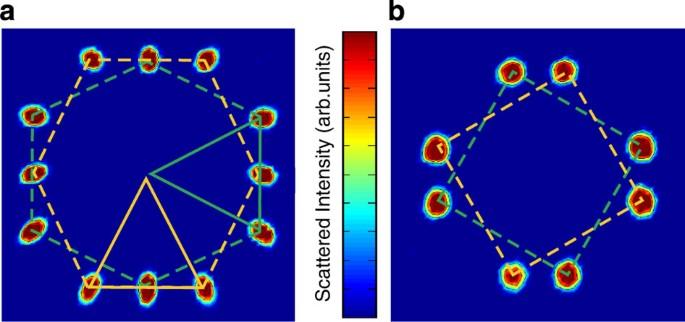Figure 1: Diffraction patterns from flux line lattices (FLLs) formed in niobium. The field direction is normal to the figure and applied parallel to a four-fold crystal axis; degenerate FLL orientations occur3,4and are indicated by the dashed polygons. (a) At ≈4.5 K and applied field ≈150 mT, the two FLLs have an isosceles triangular half-unit cell, indicated by the solid triangles. (b) At ≈2 K and ≈80 mT, there are two square FLLs tilted away from the crystal axes. The incident beam passes through the image centres, which have been masked. Figure 1: Diffraction patterns from flux line lattices (FLLs) formed in niobium. The field direction is normal to the figure and applied parallel to a four-fold crystal axis; degenerate FLL orientations occur [3] , [4] and are indicated by the dashed polygons. ( a ) At ≈4.5 K and applied field ≈150 mT, the two FLLs have an isosceles triangular half-unit cell, indicated by the solid triangles. ( b ) At ≈2 K and ≈80 mT, there are two square FLLs tilted away from the crystal axes. The incident beam passes through the image centres, which have been masked. Full size image The lattice vectors describing the two-dimensional FLL lie perpendicular to the direction of magnetic induction , and by itself each lattice vector must satisfy the HB theorem. In this study, we consider the FLL shape formed by two of these lattice vectors and find that this cannot vary smoothly with field direction . We further examine the nature of the singularities in FLL shape, which appear intriguingly different from those of a tangent vector. Singularities in FLL structure The Poincaré-Hopf theorem states that the total 'winding number' of a vector field on a surface is equal to χ , the 'Euler characteristic' of that surface [12] , [13] . We remind the reader that for a polyhedron, χ is the number of faces minus the number of edges plus the number of vertices; for a cube, χ =6−12+8=2 and it is homeomorphic to a sphere; hence, χ =2 for a sphere also. This means that a vector field on its surface must circulate around at least one singularity. 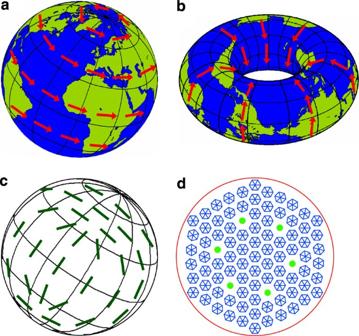Figure 2: Surface patterns of tangent objects and the hairy ball theorem. (a) Vectors on the surface of a sphere. A `w=1 singularity at the North pole is shown; (b) no singularity is necessary on the surface of a torus; (c) twofold symmetric tangent objects (lines) on the surface of a sphere. Twow=+½ singularities are shown; (d) sixw=+1/61/6 singularities (marked with filled circles) for a tangent object with sixfold symmetry. Foraandcthere would be equivalent singularities on the unseen half of the sphere. In Figure 2a , we illustrate a singularity with winding number w =+1. The value of w reflects the fact that on going around the singularity, the vector direction rotates by one full turn. The HB theorem can be satisfied on a sphere by the existence of two of these singularities, for example, westerly winds circulating around the globe except for still points at the North and South poles ( Fig. 2a ). The inevitable existence of singularities on a sphere, which affects the physics on a global scale, does not originate from the local physics, but arises from underlying geometry. For example, if the Earth were toroidal ( χ =0), winds could circulate in the same local direction everywhere ( Fig. 2b ). Figure 2: Surface patterns of tangent objects and the hairy ball theorem. ( a ) Vectors on the surface of a sphere. A ` w =1 singularity at the North pole is shown; ( b ) no singularity is necessary on the surface of a torus; ( c ) twofold symmetric tangent objects (lines) on the surface of a sphere. Two w =+½ singularities are shown; ( d ) six w =+1/61/6 singularities (marked with filled circles) for a tangent object with sixfold symmetry. For a and c there would be equivalent singularities on the unseen half of the sphere. Full size image In atmospheric physics, singularities may be realised by making the tangent vector—the wind velocity—vanish, as at the eye of a storm. In contrast, null FLL vectors are forbidden by flux quantisation, which fixes the FLL unit cell area A = Φ 0 / B . In turn, this guarantees that the pair of basis vectors describing the FLL are linearly independent. The maximal number m of continuous linearly independent vector fields that a sphere in n dimensions can support is assessable analytically [14] , [15] , [16] , [17] . For n odd, it is found that m =0, consistent with the HB theorem for n =3. As neither of the two FLL basis vectors can be continuous, the FLL shape cannot vary smoothly with field direction. Tangent vectors and FLL shapes are clearly rather different objects, and indeed, these differences are reflected in the distinctive nature of their singularities. However, the concept of 'winding number' is preserved. For tangent vectors, w must be integral (see Fig. 2a ), but tangent objects of higher symmetry can adopt a fractional w . In Figure 2c , we illustrate half-integral winding number singularities for a twofold symmetric object: a vector without an arrow. The Euler characteristic χ depends only on the surface and remains +2 for a sphere. Thus, to 'comb a ball of uprooted hairs', four w =+½ singularities are a possible solution. In Figure 2d , we consider tangent objects having sixfold symmetry, appropriate for an equilateral triangular FLL. Here, a w =+1 singularity can be 'delocalised' into six w =+1/61/6 points. Remarkably, we shall see that such singularities actually exist—in equilibrium—in nature. There are several ways by which the FLL structure can satisfy the HB theorem, one or more of which may occur in any given type-II superconductor. We examine three ways that are observed experimentally. No favoured FLL orientation The first way is trivial: no particular FLL orientation is favoured. As FLL orientation is not determined by standard approaches [1] , [2] based on 'conventional' ( s -wave) theory [18] , underlying anisotropy specific to the superconductor, even if weak, is a prerequisite to establishing any preferred FLL orientation, even when the FLL shape is a 'conventional' equilateral triangle. Any impurities present will smooth out underlying anisotropy [19] and also pin the FLL. Therefore, it is unsurprising that observations of orientationally disordered FLL's have been the preserve of situations in which impurity or pinning effects are significant. Examples include 2 H -NbSe 2 [20] , [21] , Bi 2 Sr 2 CaCu 2 O 8 [22] , the nickel borocarbide superconductors [10] , [11] and iron pnictides [23] , as well as experiments in which strong disorder is purposely introduced [24] . FLL domain formation A second way may occur when the field lies along a symmetry direction or in a symmetry plane of the superconducting crystal. Two or more degenerate FLL structures can then exist, all with the same shape but orientated differently, as permitted by the crystal symmetries. FLL domains with any one of these degenerate orientations will form in different parts of the crystal. On rotating through the symmetry position, the domain occupations will change rapidly, such that one set of FLL vectors will fade in diffracted neutron intensity, simultaneously being replaced by a differently orientated set. This is exemplified by the FLL shapes and orientations observed in high-purity Nb, a conventional, low- κ superconductor with cubic crystal structure [3] , [4] , [5] , [6] . In Figure 1a , we show the FLL observed at high temperatures for fields parallel to [001] (see Methods ). Here, the FLL half-unit cell is an isosceles triangle. This twofold shape spontaneously breaks the fourfold crystal symmetry, and two degenerate FLL domains co-exist. 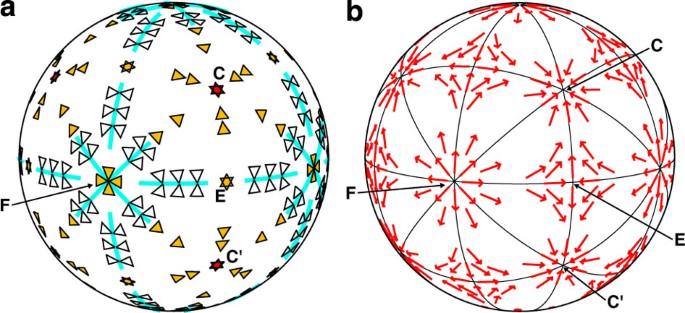Figure 3: Flux line lattice (FLL) structures and the hairy cube. (a) FLL structures observed3,5as a function of field direction in niobium under the conditions ofFigure 1a. For clarity, only one of the two triangular half-unit cells is shown, except at the <110> (E) and <111> (C and C′) directions. Isosceles half-unit cells are indicated by filled triangles, and equilateral triangles are coloured in red. Thick lines denote the field directions where two FLL domains co-exist, and across which there are sudden changes in the preferred FLL orientation. The two co-existing domains are shown on either side of the underlying crystal mirror plane (seeFig. 1afor the <100> (F) direction). (b) The projection of a 'hairy cube' onto the surface of a sphere; this is compared in the text with the structures represented ina. To understand how spontaneous symmetry breaking and domain formation help satisfy the HB theorem, we compare in Figure 3 the FLL shapes and orientations observed in Nb as a function of field direction ( Fig. 3a ), with the simplest configuration of tangent vectors on a sphere possessing cubic symmetry ( Fig. 3b ). In Figure 3b , w =+1 singularities are placed at the six cube-face (labelled 'F') axes having fourfold symmetry and also at the eight cube-corner ('C') threefold directions, whereas w =−1 singularities are placed at the 12 twofold cube-edge ('E') directions. Comparing with Figure 3a , we see that the FLL shape keeps its continuity for field directions near C by effectively 'delocalising' the singularity (see Fig. 2d ). At E, the singularity is also delocalised: by following the FLL shape as rotates in the CEC′ mirror plane, a geometric phase shift of π is seen between the equilateral triangular half-unit cells originating at C and C′, yet at E, both half-unit cells represent the same isosceles FLL. In stark contrast, a local character remains at the fourfold axis F, where two line singularities along the FC and FC′ directions intersect (see Fig. 3a ). At F, smooth distortions in FLL shape are afforded through the coexistence of multiple FLL domains of similar shape but different orientation. We point out that the FLL's geometric phase twists discontinuously as the F point is circumnavigated; rapid switches in domain occupancy are observed as crosses the FC and FC' mirror planes [5] . Figure 3: Flux line lattice (FLL) structures and the hairy cube. ( a ) FLL structures observed [3] , [5] as a function of field direction in niobium under the conditions of Figure 1a . For clarity, only one of the two triangular half-unit cells is shown, except at the <110> (E) and <111> (C and C′) directions. Isosceles half-unit cells are indicated by filled triangles, and equilateral triangles are coloured in red. Thick lines denote the field directions where two FLL domains co-exist, and across which there are sudden changes in the preferred FLL orientation. The two co-existing domains are shown on either side of the underlying crystal mirror plane (see Fig. 1a for the <100> (F) direction). ( b ) The projection of a 'hairy cube' onto the surface of a sphere; this is compared in the text with the structures represented in a . Full size image Jumps in FLL shape A third way to realise the HB theorem is by discontinuous changes in FLL shape with field direction . This behaviour is also exhibited by high-purity Nb at low temperatures (≤ 2.5 K) and fields within the intermediate mixed state. Unlike in the mixed state, in which the sample is packed with flux lines, in the intermediate mixed state, the sample contains Meissner regions of zero flux and regions of flux lines [25] , [26] . At parallel to [001] in Nb, the unit FLL cell is exactly square, but its orientation breaks the fourfold crystal symmetry, and two degenerate domains coexist ( Fig. 1b ). This square shape is observed to transform discontinuously with rotations of away from [001] [6] . Unlike in the mixed state in which flux lines interact repulsively, in the intermediate mixed state, the interaction is attractive over a range of distances [25] . It would be intriguing to determine if this change in local physics affects whether the HB theorem is satisfied by the appearance of discontinuous distortions or whether it is relieved through FLL domain formation. We conclude that spontaneous symmetry-breaking FLL structures are surprisingly likely to occur. If the FLL elects to fulfill the HB theorem by forming domains, then domain formation implies degenerate FLL orientations, which compel the FLL structure to break some underlying crystal symmetry. FLL's are sometimes dubbed 'unconventional' if they depart from the equilateral triangular prediction of standard Ginzburg–Landau theory [2] , valid for conventional ( s -wave) isotropic superconductors [18] . The HB theorem makes it clear that 'unconventional' FLL structures are not exclusive to unconventional superconductors and therefore do not necessarily imply unconventional superconductivity. Although geometry decrees that the FLL must cleave to the HB theorem, it is local physics that determines exactly how this is achieved. Clearly, the HB theorem will be seminal in stimulating FLL explorations as a function of field direction. To date, a survey of symmetry-breaking FLL's has been reported only in Nb [3] , [4] , [5] , [6] , in which intriguing FLL structures and transitions are observed at so-called 'magic' directions away from the principal crystal axes. These 'magic' directions are likely tied to corresponding features in the anisotropic Nb Fermi surface [5] , [6] . The additional asymmetries introduced by unconventional superconducting wave functions may allow new local physics to emerge. We point out that PrOs 4 Sb 12 is an alluring candidate for prospective angle-resolved FLL morphology studies. With tetrahedral ( T h ) point group symmetry and no four-fold rotation axes, PrOs 4 Sb 12 reveals a uniquely orientated, distorted triangular FLL for fields parallel to one of the a , b or c axes [27] . The HB theorem stipulates that interesting FLL transitions must occur as the field is rotated; these transitions may provide valuable information as to the hitherto unresolved nature of the PrOs 4 Sb 12 superconducting gap. Finally, we remark that it will be fascinating to ascertain which of the distinct modes are exhibited and the location of singularities on the -rotation sphere, not only in conventional and unconventional superconductors but also in any structure featuring one or more ordering vectors normal to B , such as the magnetic 'skyrmion lattice' in MnSi [28] . Small-angle neutron scattering The FLL structures of high-purity Nb, presented in this paper to illustrate the HB theorem, were measured using a double-crystal diffractometer at Oak Ridge National Laboratory [3] and small-angle neutron scattering (SANS) instruments at the Institut Laue-Langevin and the Paul Scherrer Institut [5] . In a typical SANS setup, neutrons of wavelengths ≈10 Å were collimated over a distance ≈18 m before reaching the sample. A two-dimensional area detector at a similar distance behind the sample detected the diffracted neutrons. The samples—large (≈10 g), high-purity single crystals of Nb—were mounted inside a cryomagnet providing a magnetic field approximately parallel to the incident neutron beam. A full description of the SANS measurements and sample details are contained in Laver et al . [5] , and the double-crystal diffractometer measurements are described in Christen et al . [3] The FLL diffraction patterns shown in Figure 1 depict integrated intensities, collected by rocking the Bragg diffraction spots through the Ewald sphere. As the FLL is two-dimensional, the real space arrangement is readily visualised from the reciprocal lattice vectors by rotating these diffraction images by 90° about the field axis (normal to the page in Fig. 1 ). Elemental Nb is bcc and has a low Ginzburg–Landau parameter ( κ ≃ 0.77) near T c =9.27 K. With fields B parallel to the four-fold [001] crystal axis, a cornucopia of distinct FLL structures is observed, depending on the temperature and field value [4] . In contrast, at all temperatures and fields parallel to the three-fold [111] crystal axis, a single domain of equilateral triangular FLL is observed [3] , [5] . In this paper, we pick two regions of temperature and field value that aptly show the different ways in which the HB theorem may manifest itself as the field direction is rotated relative to the crystal. The conditions for the first region are high temperatures (≤4 K); at all values of field parallel to [001], the FLL half-unit cell is an isosceles triangle, and two degenerate FLL domains coexist ( Fig. 1a ). The observed evolution of this FLL as the field is rotated is shown in Figure 3a . This figure is compiled from results unveiled in Christen et al . [3] and Laver et al . [5] For the second region, the conditions are low temperatures (≤2.5 K) and fields within the intermediate mixed state. The intermediate mixed state arises in superconductors of low κ close to 1√2, at field values close to the lower critical field and in samples with a finite demagnetisation factor [25] , [26] . Under these conditions and with parallel to [001], a square unit cell is observed with nearest-neighbour directions ≈ ± 15° from the <100> crystal directions, as shown in Figure 1b . The observed evolution with field direction of this FLL is detailed in Mühlbauer et al . [6] How to cite this article: Laver, M. et al . Magnetic flux lines in type-II superconductors and the 'hairy ball' theorem. Nat. Commun. 1:45 doi: 10.1038/ncomms1047 (2010).